Identification of ROCK1 kinase as a critical regulator of Beclin1-mediated autophagy during metabolic stress The Ser/Thr Rho kinase 1 (ROCK1) is known to have major roles in a wide range of cellular activities, including those involved in tumour metastasis and apoptosis. Here we identify an indispensable function of ROCK1 in metabolic stress-induced autophagy. Applying a proteomics approach, we characterize Beclin1, a proximal component of the phosphoinositide 3-kinase class III lipid–kinase complex that induces autophagy, as an interacting partner of ROCK1. Upon nutrient deprivation, activated ROCK1 promotes autophagy by binding and phosphorylating Beclin1 at Thr119. This results in the specific dissociation of the Beclin1–Bcl-2 complex without affecting the Beclin1–UVRAG interaction. Conversely, inhibition of ROCK1 activity increases Beclin1–Bcl-2 association, thus reducing nutritional stress-mediated autophagy. Genetic knockout of ROCK1 function in mice also leads to impaired autophagy as evidenced by reduced autophagosome formation. These results show that ROCK1 acts as a prominent upstream regulator of Beclin1-mediated autophagy and maintains a homeostatic balance between apoptosis and autophagy. Rho kinases, ROCKs, are serine/threonine kinases that were initially identified as activated Rho (Rho-GTP) interacting proteins [1] . ROCKs function as versatile kinases, phosphorylating various substrates such as myosin light chain phosphatase, LIM kinase, phosphatase and tensin homologue, insulin receptor substrate, ezrin/radixin/moesin proteins, and JNK interacting protein (JIP-3) [2] , [3] , [4] , [5] , [6] . Two ROCK isoforms exist—ROCK1 (ROKβ) and ROCK2 (ROKα). Both isoforms consist of an amino terminal kinase domain, a coiled-coil region consisting of a Rho-binding domain, a pleckstrin homology domain and a cysteine-rich domain. The isoforms share 92% homology in their kinase domain and phosphorylate a consensus motif R/KXS/T or R/KXXS/T [2] . These enzymes have a role in varied cellular processes, including cell–cell adhesion, migration, invasion, transformation, mitosis, DNA damage and apoptosis [2] , [5] , [7] , [8] . In addition, accumulating evidence strongly suggests a role of ROCK in glucose metabolism [4] , [6] , [9] , although the exact mechanisms involved remain to be elucidated. A highly conserved, regulated process of self-cannibalization to maintain cellular homeostasis and regain energy is termed ‘autophagy’. Autophagy occurs under basal conditions, for example, to degrade long-lived proteins, but is mainly induced in response to stress [10] , [11] . Under stress, such as an infection, autophagy is known to target pathogens to lysosomal degradation [12] , [13] . Conversely, during metabolic stress, autophagy provides ATP for cellular activity and preserves cell viability [14] , [15] . Metabolic stress is common in cancer cells that have outgrown their nutrient supply because proliferation outpaces angiogenesis, which provides nutrients. Under such harsh conditions, cancer cells must adapt, and they do so by inducing autophagy, a process whereby the cells ‘self-eat’ and also protect themselves from cell death. Autophagy, characterized by the formation of autophagosomes, is an orchestrated process involving several steps: initiation, nucleation, elongation, maturation and degradation. At least 15 different proteins are involved in the formation of autophagosomes [13] . Beclin1 (ATG6) is a well-conserved protein and has a central role during the autophagy process. Beclin1 was initially identified as the anti-apoptotic protein, Bcl-2, interacting partner [16] , [17] , [18] . During non-stress, normal conditions, Bcl-2 binds Beclin1 and inhibits autophagosome formation. However, upon starvation Beclin1 is released from Bcl-2 and can then proceed to perform its function in autophagy [19] , [20] . In addition, Beclin1 forms a multiprotein complex with PI(3)KC3 (Vps34) and UVRAG, a coiled-coil, ultraviolet irradiation resistance-associated gene protein, to induce autophagosome formation [21] . Beclin1-null mice are embryonic lethal, and Beclin1 heterozygous mice show a higher incidence of spontaneous tumour development [22] . In addition, Beclin1 is known to be deleted/underexpressed in several types of cancers, including breast and ovarian cancer [23] , [24] . Recently, it was reported that Beclin1, as well as UVRAG, are mutated in cancer cells with microsatellite instability [25] , [26] . These observations suggest a crucial role of Beclin1 during autophagy and tumour suppression. Related to this, ROCK1 overexpression has also been observed in a number of cancers and is associated with poor prognosis [27] , [28] , [29] . Furthermore, activating ROCK1 somatic mutations were identified in human cancers [30] . Interestingly, ROCK is known to have a major role in degradation of mutant Huntington protein via proteasome degradation and autophagy [31] . In addition, a recent report suggests a role of ROCK in autophagosome size regulation [32] . Here we identify Beclin1 as a novel ROCK1 substrate that is phosphorylated during metabolic stress. We further show that ROCK1 phosphorylates Beclin1 in its BH3 domain, allowing for Bcl-2 dissociation during nutrient stress to induce autophagy. Inhibition of ROCK1 activity leads to autophagy impairment, causing cell death in glucose-starved cancer cells. Thus, our findings identify ROCK1 as a critical regulator of metabolic stress signalling and provide new insights into its role in autophagy. Identification of Beclin1 as a ROCK1-binding partner As we hypothesized that ROCK1 may have a key role during nutrient stress, we performed co-immunoprecipitation (IP) mass spectroscopy (MS) study to identify ROCK1-interacting proteins. Endogenous ROCK1 was immunoprecipitated from HeLa cells incubated in normal (DMEM) or Hank’s balanced salt solution (HBSS; starvation) media, and the resulting precipitates were subjected to liquid chromatography MS/MS analysis. Among the several peptides that were identified as putative binding partners of ROCK1 under nutrient stress conditions, Beclin1 was of primary interest ( Fig. 1a ). Moreover, upon starvation the abundance of both Beclin1 and ROCK1 increased in the 20,000 g fraction (corresponding to endoplasmic reticulum/mitochondria) and in the 100,000 g fraction (cytosol; Supplementary Fig. S1a ). To confirm the MS results, co-IP experiments were performed in both HeLa ( Fig. 1a , right panel) and 293T ( Fig. 1b ) cells under normal (high glucose) and starved (HBSS) conditions. The interaction of Beclin1 with ROCK1 observed under normal (high glucose) conditions increased significantly during HBSS treatment. To further confirm Beclin1 interaction with ROCK1 during metabolic stress, live-cell imaging and Förster resonance energy transfer (FRET) was performed. Upon addition of HBSS, the N-terminal yellow fluorescent protein (YFP)-tagged ROCK1 associated with the cyan fluorescent protein (CFP)-tagged Beclin1 ( Fig. 1c ). In addition, confocal analysis showed that Beclin1 exhibited a diffuse cytoplasmic pattern and did not appear to colocalize with ROCK1 in the presence of glucose. However, when the cells were starved, Beclin1 translocated to the perinuclear region and was observed in close proximity to ROCK1 ( Supplementary Fig. S1b ). All of these results suggested that ROCK1 interacts with Beclin1 in response to nutrient starvation. 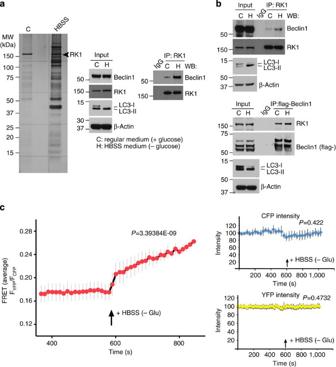Figure 1: Functional interaction of Beclin1 with ROCK1 upon metabolic stress. (a) Identification of Beclin1 as a substrate of ROCK1 via affinity purification. Left panel: HeLa cells growing in control (C: nutrient-rich media) or starved in HBSS (H) for 4 h were lysed and subjected to IP with ROCK1 cross-linked beads. Proteins bound were eluted and detected by SDS–PAGE, followed by silver staining that presents precipitated proteins identified by LC-MS/MS. Right panel: HeLa cells grown in control media or HBSS (4 h) were collected, whole cell lysates prepared and immunoprecipitated with ROCK1 cross-linked beads. The resulting immune complexes were divided into two, and were subjected to SDS–PAGE and analysed for Beclin1 (MES buffer) and ROCK1 (MOPS buffer). Inputs and IP were analysed by western blotting. HBSS-treated cell extracts were used for IgG IP controls. Whole cell lysates (10%) were run for inputs. Total cell lysates were rerun and analysed for LC3 and β-actin. (b) Co-IP was performed with 293T whole cell extracts by using ROCK1-crosslinked agarose, and the resulting IP was blotted with indicated antibodies. 293T cells transfected with Flag-Beclin1 for 36 h, cultured in control media or starved (4 h), were immunoprecipitated with anti-Flag beads. Inputs and immune complexes were resolved and detected. Total cell lysates were rerun and examined for LC3 and β-actin expression. (c) Interaction of YFP-ROCK1 and CFP-Beclin1 was examined by using live cell spinning disk microscopy and FRET in live cells. Graph represents FRETAverageratio changes (YFP-ROCK1/CFP-Beclin1) upon starvation. Data represents mean±s.e.m.;n=6. Three different experiments were performed. For the control, the right top graph represents CFP intensity over time (corrected for photobleach), and the right bottom right represents YFP intensity (corrected for photobleach). In both control FRET experiments, no significant change was observed in fluorescence, in the presence or absence of HBSS medium.Pvalues were calculated using Student'st-test. Figure 1: Functional interaction of Beclin1 with ROCK1 upon metabolic stress. ( a ) Identification of Beclin1 as a substrate of ROCK1 via affinity purification. Left panel: HeLa cells growing in control (C: nutrient-rich media) or starved in HBSS (H) for 4 h were lysed and subjected to IP with ROCK1 cross-linked beads. Proteins bound were eluted and detected by SDS–PAGE, followed by silver staining that presents precipitated proteins identified by LC-MS/MS. Right panel: HeLa cells grown in control media or HBSS (4 h) were collected, whole cell lysates prepared and immunoprecipitated with ROCK1 cross-linked beads. The resulting immune complexes were divided into two, and were subjected to SDS–PAGE and analysed for Beclin1 (MES buffer) and ROCK1 (MOPS buffer). Inputs and IP were analysed by western blotting. HBSS-treated cell extracts were used for IgG IP controls. Whole cell lysates (10%) were run for inputs. Total cell lysates were rerun and analysed for LC3 and β-actin. ( b ) Co-IP was performed with 293T whole cell extracts by using ROCK1-crosslinked agarose, and the resulting IP was blotted with indicated antibodies. 293T cells transfected with Flag-Beclin1 for 36 h, cultured in control media or starved (4 h), were immunoprecipitated with anti-Flag beads. Inputs and immune complexes were resolved and detected. Total cell lysates were rerun and examined for LC3 and β-actin expression. ( c ) Interaction of YFP-ROCK1 and CFP-Beclin1 was examined by using live cell spinning disk microscopy and FRET in live cells. Graph represents FRET Average ratio changes (YFP-ROCK1/CFP-Beclin1) upon starvation. Data represents mean±s.e.m. ; n =6. Three different experiments were performed. For the control, the right top graph represents CFP intensity over time (corrected for photobleach), and the right bottom right represents YFP intensity (corrected for photobleach). In both control FRET experiments, no significant change was observed in fluorescence, in the presence or absence of HBSS medium. P values were calculated using Student's t -test. Full size image ROCK1 activity is essential for interaction with Beclin1 To determine whether ROCK1 activity was necessary for Beclin1 interaction, cells were treated with a well-established Rho kinase inhibitor, Y27632, and endogenous ROCK1 or Beclin1 was pulled down in the presence or absence of HBSS. Similar to results in Fig. 1a , Beclin1 binding to ROCK1 increased upon starvation in non-treated cells ( Fig. 2a ). However, in Y27632-treated cells, this interaction was significantly decreased. This result suggests that ROCK1 activity is needed for Beclin1 interaction. To test whether ROCK1 activity increased upon glucose starvation, we performed an in vitro kinase assay with ROCK1 immunoprecipitated from HeLa and EJ cells grown in the presence of HBSS for various time points utilizing MYPT1, a known substrate of ROCK1. As shown in Fig. 2b , ROCK1 from starved cells was able to phosphorylate MYPT1 efficiently as compared with ROCK1 from control cells (non-starved). Moreover, endogenous ROCK activity was upregulated upon starvation as seen by increase in P-MYPT1 ( Fig. 2c ). In addition, ROCK activity increased significantly upon metabolic stress in cancer and non-cancer cell lines, as observed by enzyme-linked immunosorbent assay, using MYPT1 as a substrate ( Fig. 2d and Supplementary Fig. S2 ). Next, to examine whether increase in ROCK1 activity depended on Beclin1 interaction, we determined ROCK1 activity in Beclin1 knockdown cells upon starvation. As shown in Fig. 2e (left panel), Beclin1 was efficiently knocked down in HeLa cells; however, there was no downregulation of ROCK activity. These data suggest that Beclin1 interaction with ROCK1 is downstream of increase in ROCK activity. 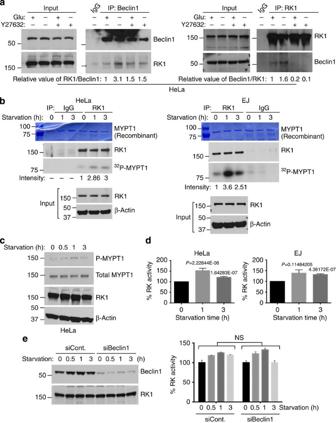Figure 2: ROCK1 is activated upon metabolic stress. (a) Inhibition of ROCK1 activity ablates the interaction between Beclin1 and ROCK1. HeLa cells were untreated (H2O) or treated with 10 μM ROCK1 inhibitor, Y27632, for 8 h and then cultured in control media (+) or HBSS (−) for 4 h. Cells were collected, lysed and immunoprecipitated with Beclin1 (left panel) or ROCK1 (right panel) antibody. Left panel: immune complexes were divided into two (ROCK1-MOPS buffer and Beclin1-MES buffer) and probed for ROCK1 and Beclin1. Relative values of ROCK1 versus Beclin1 are shown. (b) An increase in ROCK1-mediated phosphorylation of MYPT1 upon starvation. HeLa and EJ cells were starved in HBSS for indicated time points and endogenous ROCK1 was immunoprecipitated. Anin vitrokinase assay was performed using MYPT1 as substrate and immune-complexed ROCK1. Proteins were resolved and visualized with Coomassie staining (top), western blot analysis (middle) and autoradiography (bottom). Inputs were examined for ROCK1 and β-actin. (c) HeLa cells incubated in HBSS were collected and endogenous phosphorylation of MYPT1 was determined by western blotting. The same blot was then washed in TBST for 30 min, blocked in 5% milk and was analysed for total MYPT1 as a control. Extracts from this experiment were rerun on 7.5% gel and analysed for ROCK1 and β-actin. (d) ROCK activity is increased upon starvation. Cell lines (HeLa and EJ) grown in control (+Glu) or starved with HBSS for 1 and 3 h were lysed, extracts normalized and ROCK kinase activity was measured by performing enzyme-linked immunosorbent assay. Graphs represent ROCK activity in starved cells plotted as percent of ROCK1 activity in control (glucose-rich) cells. Data were obtained from triplicates performed at the same time (mean±s.d.).P-value was calculated using Student’st-test. (e) ROCK1 activity is not dependent on Beclin1. siControl (siCont.) and siBeclin1 knockdown cells were incubated in starvation media (HBSS) for indicated time. Resulting cell extracts were used to confirm Beclin1 knockdown and ROCK1 expression (left panel). Cell extracts from the same experiment were used for enzyme-linked immunosorbent assay measuring ROCK activity (right panel). Graph represents mean±s.d. of duplicate samples read at the same time (Student’st-test; NS, not significant). Figure 2: ROCK1 is activated upon metabolic stress. ( a ) Inhibition of ROCK1 activity ablates the interaction between Beclin1 and ROCK1. HeLa cells were untreated (H 2 O) or treated with 10 μM ROCK1 inhibitor, Y27632, for 8 h and then cultured in control media (+) or HBSS (−) for 4 h. Cells were collected, lysed and immunoprecipitated with Beclin1 (left panel) or ROCK1 (right panel) antibody. Left panel: immune complexes were divided into two (ROCK1-MOPS buffer and Beclin1-MES buffer) and probed for ROCK1 and Beclin1. Relative values of ROCK1 versus Beclin1 are shown. ( b ) An increase in ROCK1-mediated phosphorylation of MYPT1 upon starvation. HeLa and EJ cells were starved in HBSS for indicated time points and endogenous ROCK1 was immunoprecipitated. An in vitro kinase assay was performed using MYPT1 as substrate and immune-complexed ROCK1. Proteins were resolved and visualized with Coomassie staining (top), western blot analysis (middle) and autoradiography (bottom). Inputs were examined for ROCK1 and β-actin. ( c ) HeLa cells incubated in HBSS were collected and endogenous phosphorylation of MYPT1 was determined by western blotting. The same blot was then washed in TBST for 30 min, blocked in 5% milk and was analysed for total MYPT1 as a control. Extracts from this experiment were rerun on 7.5% gel and analysed for ROCK1 and β-actin. ( d ) ROCK activity is increased upon starvation. Cell lines (HeLa and EJ) grown in control (+Glu) or starved with HBSS for 1 and 3 h were lysed, extracts normalized and ROCK kinase activity was measured by performing enzyme-linked immunosorbent assay. Graphs represent ROCK activity in starved cells plotted as percent of ROCK1 activity in control (glucose-rich) cells. Data were obtained from triplicates performed at the same time (mean±s.d.). P -value was calculated using Student’s t -test. ( e ) ROCK1 activity is not dependent on Beclin1. siControl (siCont.) and siBeclin1 knockdown cells were incubated in starvation media (HBSS) for indicated time. Resulting cell extracts were used to confirm Beclin1 knockdown and ROCK1 expression (left panel). Cell extracts from the same experiment were used for enzyme-linked immunosorbent assay measuring ROCK activity (right panel). Graph represents mean±s.d. of duplicate samples read at the same time (Student’s t -test; NS, not significant). Full size image ROCK1 was initially identified as an effector of RhoA-GTPase and is activated by RhoA-GTP under several conditions [1] , [33] . To determine, whether increased ROCK1 activity upon metabolic stress is due to RhoA-GTP, we performed active RhoA assay. Rhotekin-binding assay was performed using cell lysates from HeLa cells incubated in DMEM or HBSS. We did not observe an increase in active RhoA upon metabolic stress, suggesting that increase in ROCK1 activity was independent of RhoA ( Supplementary Fig. S3a ). ROCK1 cleavage and activation by caspase-3 has been well documented under certain stress conditions [34] . However, no significant ROCK1 cleavage was observed during nutritional stress ( Fig. 2c ). Another family of Rho-GTPase, RhoE, is also known to regulate ROCK1 activity [35] . Therefore, we examined RhoE levels upon glucose starvation. As shown in Supplementary Fig. S3b , RhoE was upregulated in starved HeLa cells. To determine whether ROCK1 activity was regulated by RhoE during metabolic stress, we next knocked down RhoE ( Supplementary Fig. S3b ) and incubated these cells in DMEM or HBSS media. RhoE knockdown increased ROCK activity upon starvation ( Supplementary Fig. S3c ), suggesting that RhoE may negatively regulate ROCK1. This result is consistent with previous reports that show RhoE, unlike RhoA, can regulate ROCK1 in a negative manner [35] . Taken together, these results indicate that the increase of ROCK1 activity upon metabolic stress is independent of RhoA and is required for Beclin1 interaction. ROCK1 activity is required for starvation-induced autophagy As Beclin1 is a proximal component in the autophagy machinery, we examined the role of ROCK1 during nutritional stress-induced autophagy. To do so, we monitored lipidated LC3 (LC3II) levels, which are known to correlate with autophagosome formation [36] . ROCK1 −/− mouse embryonic fibroblasts (MEFs) were compared with wild-type (WT) MEFs in HBSS media. Upon starvation, WT MEFs showed an increase in LC3II, as well as an increase in LC3 punctae determined by immunofluorescence ( Fig. 3a ). However, ROCK1 −/− MEFs exhibited a significant decrease in LC3 punctae ( Fig. 3a ), suggesting ROCK1 is essential for efficient autophagy process. In addition, using short hairpin RNA (shROCK1-#1), as well as siROCK1-#2 and siROCK1-#3, we observed specific knockdown of ROCK1 ( Fig. 3b ), without affecting ROCK2 levels ( Supplementary Fig. S4a ). Levels of processed LC3 (LC3II) in EJ cells grown in glucose-rich media were low as compared with cells that were nutrient deprived (HBSS) ( Fig. 3b , left panel). Conversely, LC3 processing was not observed following nutrient deprivation if ROCK1 was silenced ( Fig. 3b , left panel). Similarly, small interfering RNA-mediated suppression of ROCK1 in HeLa cells reduced lipidated LC3 levels upon starvation ( Fig. 3b , right panel, and Supplementary Fig. S4a ). It is known that LC3II on autophagosomes is degraded upon autophagosome and lysosome fusion [37] . Therefore, to assess autophagic flux, Bafilomycin A1, a drug that inhibits this fusion and thus prevents autophagic vacuole maturation [38] , was used. Similar to that in previous experiments, Y27632 treatment inhibited the accumulation of LC3II upon metabolic stress in HeLa cells ( Fig. 3c ), in the presence of Bafilomycin A1. Furthermore, p62, a multifunctional adaptor protein that is cleared by autophagy [39] , accumulated in Y27632-treated cells ( Supplementary Fig. S4b ). To further examine autophagic flux, we used DQ Red BSA, which is labelled with a self-quenched red fluorescent dye and can emit fluorescence upon lysosomal protease cleavage. As shown in Supplementary Fig. S5 , we observed a significant increase in dequenched DQ Red BSA-labelled vesicles colocalizing with GFP-LC3 punctae in control-starved cells, but not in Y27632-treated cells. This suggests that inhibition of ROCK1 suppresses autophagosome formation directly, rather than by interfering with lysosomal activity, thus affecting autophagic flux. We further investigated whether ROCK1 has a role in autophagy by examining the morphological features of endogenous LC3 (seen as punctae). HeLa cells left untreated or treated with the ROCK inhibitor Y27632 were cultured in HBSS media, and the patterns of LC3 punctae were analysed by immunofluorescence. 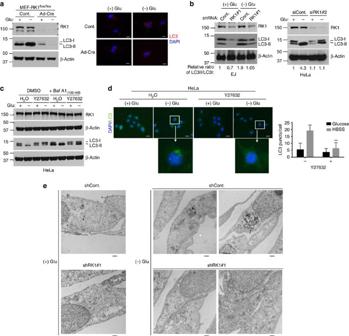Figure 3: ROCK1 activity is essential for metabolic stress-induced autophagy. (a) The effect of ROCK1 depletion on autophagy marker, LC3II. MEF ROCK1flox/floxcells were generated and treated with Con or Ad-Cre for 72 h. Cells were then incubated in nutrient-rich (+Glucose) or HBSS media for 2 h. Cell extracts were resolved by SDS–PAGE and ROCK1 KO was confirmed by western blotting (left panel). The same blot was used for LC3 and β-actin expression. Cells from the same experiment were fixed with chilled acetone and immunofluroscence was performed against endogenous LC3 (red). Blue represents nuclear DAPI staining. Scale bar, 20 μm. (b) EJ cells (left) with a stable knockdown using shCont. or shROCK1#1 were incubated in control (+glucose) or nutrient-free (HBSS) medium (−glucose) for 24 h and lysed. Lysates were subjected to western blotting with antibodies indicated. HeLa cells (right) with a transient knockdown using siCont. and siROCK1#2 for 30 h were further incubated in control or HBSS media for 8 h. Whole cell extracts were prepared, resolved by SDS–PAGE and analysed for ROCK1, LC3 and β-actin. Relative ratios of LC3II/LC3I are shown. (c) HeLa cells were treated with H2O or 10 μM ROCK1 inhibitor, Y27632, for 8 h. Cells were then cultured in high glucose (0 h) or starved for in HBSS nutrient-free media for 6 h. One hour before collection, cells were incubated in dimethylsulphoxide (control) or 0.1 μM bafilomycin-A1. Whole cell lysates were resolved by SDS–PAGE and were analysed by western blotting with indicated antibodies. (d) HeLa cells incubated with H2O or 10 μM Y27632 for 8 h were washed with PBS and cultured in control (+Glu) or HBSS media (−Glu) for an additional 8 h. Cells were fixed in acetone and immunofluorescence was performed against endogenous LC3 antibody (green). Scale bar, 20 μm. Graph represents % of LC3 punctae/cell (mean±s.d.),n=25 cells; (Student’st-test) **P=0.00041. (e) Transmission electron micrographs of EJ cells with stable shCont. or shROCK1#1 knockdown, cultured in control or HBSS medium for 16 h. Arrow bars indicate autophagic vacuoles. Scale bar, 500 nm. Figure 3d shows an increase in LC3 punctae upon starvation in control cells in the absence of Y27632. However, the addition of Y27632 significantly impaired LC3 punctae formation upon nutrient stress ( Fig. 3d ). In addition, EJ cells with ROCK1 knockdown and shControl (shCont.). were stably transfected with GFP-LC3 and subjected to starvation. In shCont.-transfected EJ cells, GFP-LC3 punctae were significantly induced upon starvation, indicating upregulated autophagy ( Supplementary Fig. S4c ). However, in shROCK1#1 cells, GFP-LC3 punctae were markedly decreased under stress conditions ( Supplementary Fig. S4c ). To further confirm that ROCK1 is required for autophagy, starved EJ cells with shCont. or shROCK1#1 were examined via transmission electron microscopy to detect autophagosome formation ( Fig. 3e ). Consistent with our evidence that LC3 cleavage is highly compromised in shROCK1 cells, we observed a defect in autophagosome/autolysosome formation in these cells. Figure 3: ROCK1 activity is essential for metabolic stress-induced autophagy. ( a ) The effect of ROCK1 depletion on autophagy marker, LC3II. MEF ROCK1 flox/flox cells were generated and treated with Con or Ad-Cre for 72 h. Cells were then incubated in nutrient-rich (+Glucose) or HBSS media for 2 h. Cell extracts were resolved by SDS–PAGE and ROCK1 KO was confirmed by western blotting (left panel). The same blot was used for LC3 and β-actin expression. Cells from the same experiment were fixed with chilled acetone and immunofluroscence was performed against endogenous LC3 (red). Blue represents nuclear DAPI staining. Scale bar, 20 μm. ( b ) EJ cells (left) with a stable knockdown using shCont. or shROCK1#1 were incubated in control (+glucose) or nutrient-free (HBSS) medium (−glucose) for 24 h and lysed. Lysates were subjected to western blotting with antibodies indicated. HeLa cells (right) with a transient knockdown using siCont. and siROCK1#2 for 30 h were further incubated in control or HBSS media for 8 h. Whole cell extracts were prepared, resolved by SDS–PAGE and analysed for ROCK1, LC3 and β-actin. Relative ratios of LC3II/LC3I are shown. ( c ) HeLa cells were treated with H 2 O or 10 μM ROCK1 inhibitor, Y27632, for 8 h. Cells were then cultured in high glucose (0 h) or starved for in HBSS nutrient-free media for 6 h. One hour before collection, cells were incubated in dimethylsulphoxide (control) or 0.1 μM bafilomycin-A1. Whole cell lysates were resolved by SDS–PAGE and were analysed by western blotting with indicated antibodies. ( d ) HeLa cells incubated with H 2 O or 10 μM Y27632 for 8 h were washed with PBS and cultured in control (+Glu) or HBSS media (−Glu) for an additional 8 h. Cells were fixed in acetone and immunofluorescence was performed against endogenous LC3 antibody (green). Scale bar, 20 μm. Graph represents % of LC3 punctae/cell (mean±s.d. ), n =25 cells; (Student’s t -test) ** P =0.00041. ( e ) Transmission electron micrographs of EJ cells with stable shCont. or shROCK1#1 knockdown, cultured in control or HBSS medium for 16 h. Arrow bars indicate autophagic vacuoles. Scale bar, 500 nm. Full size image Next we investigated whether impaired autophagy due to loss of ROCK1 affected cell viability. Inhibition of ROCK1 activity during starvation resulted in a significantly decreased cell viability (shROCK1 ~1.9-fold; Y27632 ~1.96-fold) as compared with that of control (glucose fed) HeLa or EJ cells ( Supplementary Fig. S6 , left panels). In addition, as evidenced by Alamar blue cell death assay ( Supplementary Fig. S6a , right panel), ROCK1 stable knockdown in EJ cells led to increased loss in cell viability. Moreover, although TUNEL staining of siCont.-transfected HeLa cells after nutrient starvation showed 36.3% positive cells, siROCK1-transfected cells had 90.6% TUNEL-positive cells under the same experimental conditions ( Supplementary Fig. S6b , right panel). Taken together, these results indicate that ROCK1 activity is essential for functional autophagy and that impairment of ROCK1-mediated autophagy can increase cell death at early time points. Beclin1 is phosphorylated by ROCK1 at T119 As ROCK1 is a Ser/Thr kinase and ROCK1 binding to Beclin1 is enhanced upon glucose starvation, we hypothesized that Beclin1 is a direct substrate of ROCK1 in response to nutrient deprivation. To determine whether Beclin1 would be phosphorylated under these conditions, endogenous Beclin1 was immunoprecipitated from fed or starved cells, and was immunoblotted with anti-phospho Ser/Thr. As shown in Fig. 4a (lane 2), Beclin1 indeed was phosphorylated after glucose starvation, whereas the ROCK inhibitor Y27632 blocked this phosphorylation (lane 4). Similar results were obtained upon ROCK1 knockdown ( Supplementary Fig. S7a ). The phosphorylation of Flag-tagged Beclin1 purified from HeLa cell extracts or recombinant Beclin1 was measured in vitro following incubation with recombinant ROCK1. Full-length recombinant His-Beclin1 ( Supplementary Fig. S7b ) was phosphorylated by recombinant ROCK1, and this phosphorylation was blocked by Y27632 ( Fig. 4b ). Similarly, when Flag-Beclin1 purified from HeLa cell extracts was incubated with ROCK1, we observed ROCK1-mediated phosphorylation of Beclin1 as visualized by 32 P autoradiogram. This phosphorylation was a direct result of ROCK1 kinase activity, as the addition of Y27632 significantly inhibited 32 P incorporation. These data suggested that Beclin1 phosphorylation induced by starvation is likely ROCK1 dependent. Next we prepared a series of partially overlapping Flag fusion fragments of Beclin1 spanning the entire length of the Beclin1 protein. These various Flag-Beclin1 fragments (comprising residues: 1–242, 151–241 and 243–450) were tested as possible substrates for ROCK1 ( Fig. 4c ). Of the Beclin1 fragments, only Flag-Beclin1 1–242 (comprising the N-terminal 242 amino acid of Beclin1) was strongly phosphorylated by recombinant ROCK1 ( Fig. 4c ). Further exploration of Beclin1 1–242 fragment for the consensus sequence of ROCK1 substrate, R/KXS/T or R/KXXS/T, identified several putative ROCK1 phosphorylation sites. Using the Kinexus PhosphoNET kinase predictor ( http://www.phosphonet.ca ), potential ROCK1 sites were narrowed down to Ser22, Thr38 and Thr119 ( Supplementary Fig. S8 ). Mutational analyses of ROCK1 consensus sites identified that a mutant form of Flag-Beclin1 1–242, harbouring a threonine to alanine substitution at Thr119 (Flag-Beclin1 T119A), was not phosphorylated by ROCK1 ( Fig. 4d ). To further confirm that endogenous Beclin1 was phosphorylated at T119 and this site phosphorylation depended on ROCK1, we used a phospho-specific antibody against this site. We first confirmed the specificity of this antibody by using Flag-Beclin1 T119A mutant ( Fig. 4e ). As shown in Fig. 4e , starvation induced Flag-Beclin1 WT phosphorylation at T119, and this stress-induced phosphorylation was decreased upon addition of ROCK inhibitor, Y27632. However, we did not see any phosphorylation of T119A mutant upon starvation. We further confirmed whether ROCK1 could phosphorylate endogenous Beclin1 at T119 using Myc-ROCK1 WT, CA (constitutively active) or DN (dominant negative) transfected cells ( Supplementary Fig. S9 ). Endogenous Beclin1 immunoprecipitated from ROCK1 CA-transfected cells was highly phosphorylated at T119. In comparison, Beclin1 T119 phosphorylation was significantly suppressed in ROCK1 DN-transfected cells ( Supplementary Fig. S9 ). Thus, these results strongly suggest that ROCK1 can directly phosphorylate Beclin1 at T119 under nutritional stress. 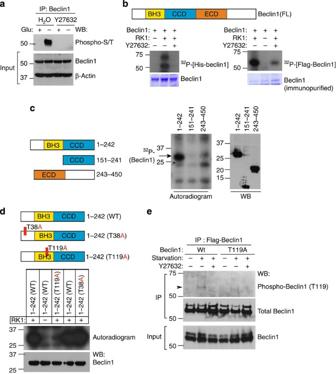Figure 4: Metabolic stress induces Beclin1 phosphorylation by ROCK1. (a) Inhibition of ROCK1 kinase activity prevents metabolic stress-mediated phosphorylation of Beclin1. HeLa cells left untreated or treated with a ROCK1 inhibitor, Y27632 (10 μM), were starved of glucose (4 h) as indicated, and endogenous Beclin1 was immunoprecipitated and blotted against phospho-Ser/Thr antibody. Whole cell lysates were run as inputs for Beclin1 and β-actin. (b) Phosphorylation of Beclin1 by ROCK1. Recombinant ROCK1 was used forin vitrokinase assay in the presence or absence of Y27632, using recombinant His-Beclin1 (left) or Flag-Beclin1 immunopurified from transfected HeLa cells (right). Proteins were resolved by SDS–PAGE; phosphorylated protein was visualized with autoradiography, and Beclin1 by Coomassie staining. (c) Identification of ROCK1-mediated phosphorylation domains in Beclin1. The indicated Flag-Beclin1 fragments were purified from HeLa cells and used as substrates forin vitroROCK1 kinase assay.32P-autoradiogram (centre) analysed phosphorylation and western blotting (WB; right) determined protein levels. Schematic representation of Beclin1 domain structure and deletion constructs are shown (left). (d) Identification of the phosphorylation site on Beclin1. Representation of point mutations in the different domains of Beclin1 are shown (left).In vitrokinase assay using Flag-Beclin1 WT and mutants (T38A and T119A), immunoprecipitated from transfected HeLa cells, as substrate and recombinant ROCK1 was performed. Phosphorylation was detected by32P-autoradiogram, and Flag-Beclin1 levels were examined by WB. (e) Flag-Beclin1 Wt or T119A transfected HeLa cells were incubated in glucose-rich or nutrient-free (HBSS) media, in the presence or absence of ROCK1 inhibitor Y27632. Total cell extracts were used for IP using Flag agarose. Eluted protein was analysed by WB against phospho-T119 (Beclin) antibody and Beclin1. Input for Beclin1 was run on 7.5% gel and immunoblotted. Figure 4: Metabolic stress induces Beclin1 phosphorylation by ROCK1. ( a ) Inhibition of ROCK1 kinase activity prevents metabolic stress-mediated phosphorylation of Beclin1. HeLa cells left untreated or treated with a ROCK1 inhibitor, Y27632 (10 μM), were starved of glucose (4 h) as indicated, and endogenous Beclin1 was immunoprecipitated and blotted against phospho-Ser/Thr antibody. Whole cell lysates were run as inputs for Beclin1 and β-actin. ( b ) Phosphorylation of Beclin1 by ROCK1. Recombinant ROCK1 was used for in vitro kinase assay in the presence or absence of Y27632, using recombinant His-Beclin1 (left) or Flag-Beclin1 immunopurified from transfected HeLa cells (right). Proteins were resolved by SDS–PAGE; phosphorylated protein was visualized with autoradiography, and Beclin1 by Coomassie staining. ( c ) Identification of ROCK1-mediated phosphorylation domains in Beclin1. The indicated Flag-Beclin1 fragments were purified from HeLa cells and used as substrates for in vitro ROCK1 kinase assay. 32 P-autoradiogram (centre) analysed phosphorylation and western blotting (WB; right) determined protein levels. Schematic representation of Beclin1 domain structure and deletion constructs are shown (left). ( d ) Identification of the phosphorylation site on Beclin1. Representation of point mutations in the different domains of Beclin1 are shown (left). In vitro kinase assay using Flag-Beclin1 WT and mutants (T38A and T119A), immunoprecipitated from transfected HeLa cells, as substrate and recombinant ROCK1 was performed. Phosphorylation was detected by 32 P-autoradiogram, and Flag-Beclin1 levels were examined by WB. ( e ) Flag-Beclin1 Wt or T119A transfected HeLa cells were incubated in glucose-rich or nutrient-free (HBSS) media, in the presence or absence of ROCK1 inhibitor Y27632. Total cell extracts were used for IP using Flag agarose. Eluted protein was analysed by WB against phospho-T119 (Beclin) antibody and Beclin1. Input for Beclin1 was run on 7.5% gel and immunoblotted. Full size image ROCK1 phosphorylates Beclin1 to disrupt Bcl-2 association T119 lies in the ROCK1 consensus motif and is highly conserved among species ( Supplementary Fig. S8 ). Moreover, it was previously reported that this site resides in the BH3 domain and, therefore, we reasoned that it might contribute to Beclin1–Bcl-2 interaction [40] , [41] . To test whether ROCK1 phosphorylation of Beclin1 was indispensable for its dissociation from Bcl-2, we performed IP experiments. Beclin1 binding to Bcl-2 was inhibited upon starvation in HeLa cells, as compared with glucose-fed control cells ( Fig. 5a ). However, Y27632 treatment significantly increased Beclin1 binding to Bcl-2 by approximately fourfold in high glucose conditions and maintained a similar level of association between Bcl-2 and Beclin1 upon HBSS starvation ( Fig. 5a ). Similar results were obtained with EJ shCont. and shROCK1 stable transfectants ( Fig. 5a ), and HeLa siCont. and siROCK1#2 ( Supplementary Fig. S10b ), confirming that ROCK1 was required for Beclin1/Bcl-2 uncoupling for autophagy to proceed during starvation. To determine whether ROCK1 phosphorylation of Beclin1 was necessary for its interaction with other binding partners in the Beclin1 core complex, Vps34 and UVRAG proteins were examined. As shown in Supplementary Fig. S10c , similar levels of Vps34 and UVRAG were pulled down in the presence or absence of Y27632. These results indicate that ROCK1 phosphorylates Beclin1 at Thr119, and this phosphorylation disrupts the Beclin1/Bcl-2 complex without affecting other Beclin1 binding partners, such as Vps34 and UVRAG, during the autophagy process. 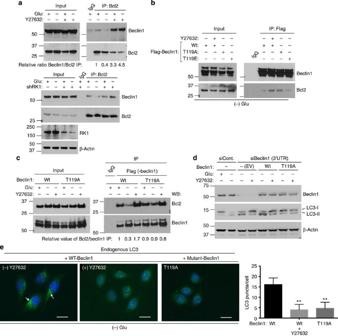Figure 5: ROCK1 phosphorylation of Beclin1 at T119 promotes Bcl-2 dissociation. (a) Inhibiting ROCK1 activity increases the association between Beclin1 and Bcl-2. HeLa cells, untreated or treated with 10 μM Y27632 (top panel), were cultured in control or glucose-free (4 h) medium, lysed and cell extracts prepared. Endogenous Bcl-2 was immunoprecipitated with cross-linked Bcl-2 agarose and resulting eluted immune complexes were resolved by SDS–PAGE and blotted against indicated antibodies. EJ shCont. and shROCK1#1 cells (bottom panel) were grown in control or starvation media for 4 h and Bcl-2 IP was performed as above. Inputs were rerun to confirm ROCK1 knockdown. (b) HeLa cells were transfected with full-length constructs of Flag-Beclin WT, Flag-Beclin T119A or Flag-Beclin T119E. Flag-Beclin WT cells were then treated with Y27632 for 8 h. Post transfection and treatment with Y27632, cells were starved in HBSS medium for 4 h, after which cells were collected and whole cell lysates prepared. IP with Flag-agarose was performed for 2 h and proteins bound to beads were eluted and used for western blotting. (c) Flag-Beclin1 Wt or T119A transfected HeLa cells were incubated in glucose-rich or nutrient-free (HBSS) media, in the presence or absence of ROCK1 inhibitor Y27632. Total cell extracts were used for IP using Flag agarose. Eluted protein was analysed by western blotting against Bcl-2 and Beclin1. Inputs and IP were run on separate gels and same exposure is shown. (d) HeLa cells with a transient knockdown using siCont. and siBeclin1–3′-untranslated region for 30 h were further left untreated or treated with 10 μM Y27632. Cells were then incubated in control or HBSS media for 8 h. Whole cell extracts were prepared, resolved by SDS–PAGE and were analysed for Beclin1, LC3 and β-actin. (e) Endogenous LC3 staining in WT- or T119A-Beclin1-transfected cells. HeLa cells transfected with Flag-Beclin WT (±Y27632) and T119A were cultured in HBSS media for 6 h, fixed with cold acetone and endogenous LC3 immunofluorescence was performed. Representative images are shown; scale bar, 20 μm. Arrows indicate punctate LC3 staining. Graph represents mean±s.d.,n=25, LC3 puncta/cell. Figure 5: ROCK1 phosphorylation of Beclin1 at T119 promotes Bcl-2 dissociation. ( a ) Inhibiting ROCK1 activity increases the association between Beclin1 and Bcl-2. HeLa cells, untreated or treated with 10 μM Y27632 (top panel), were cultured in control or glucose-free (4 h) medium, lysed and cell extracts prepared. Endogenous Bcl-2 was immunoprecipitated with cross-linked Bcl-2 agarose and resulting eluted immune complexes were resolved by SDS–PAGE and blotted against indicated antibodies. EJ shCont. and shROCK1#1 cells (bottom panel) were grown in control or starvation media for 4 h and Bcl-2 IP was performed as above. Inputs were rerun to confirm ROCK1 knockdown. ( b ) HeLa cells were transfected with full-length constructs of Flag-Beclin WT, Flag-Beclin T119A or Flag-Beclin T119E. Flag-Beclin WT cells were then treated with Y27632 for 8 h. Post transfection and treatment with Y27632, cells were starved in HBSS medium for 4 h, after which cells were collected and whole cell lysates prepared. IP with Flag-agarose was performed for 2 h and proteins bound to beads were eluted and used for western blotting. ( c ) Flag-Beclin1 Wt or T119A transfected HeLa cells were incubated in glucose-rich or nutrient-free (HBSS) media, in the presence or absence of ROCK1 inhibitor Y27632. Total cell extracts were used for IP using Flag agarose. Eluted protein was analysed by western blotting against Bcl-2 and Beclin1. Inputs and IP were run on separate gels and same exposure is shown. ( d ) HeLa cells with a transient knockdown using siCont. and siBeclin1–3′-untranslated region for 30 h were further left untreated or treated with 10 μM Y27632. Cells were then incubated in control or HBSS media for 8 h. Whole cell extracts were prepared, resolved by SDS–PAGE and were analysed for Beclin1, LC3 and β-actin. ( e ) Endogenous LC3 staining in WT- or T119A-Beclin1-transfected cells. HeLa cells transfected with Flag-Beclin WT (±Y27632) and T119A were cultured in HBSS media for 6 h, fixed with cold acetone and endogenous LC3 immunofluorescence was performed. Representative images are shown; scale bar, 20 μm. Arrows indicate punctate LC3 staining. Graph represents mean±s.d., n =25, LC3 puncta/cell. Full size image To determine whether the loss of phosphorylation at Thr119 could recapitulate inhibition of ROCK1 kinase activity during metabolic stress, we generated and compared Bcl-2 binding activity of WT, T119A (phospho-mutant) and T119E (phospho-mimetic) mutant forms of Beclin1. HeLa cells transfected with a Flag-Beclin1 WT construct in the presence of HBSS showed only slight Bcl-2/Beclin1 interaction ( Fig. 5b , lane 1). Furthermore, inhibition of ROCK1 activity by Y27632 significantly increased the binding of Bcl-2 to Beclin1, as expected ( Fig. 5b , lane 2). In agreement, Beclin1-T119A mutant pulled down endogenous Bcl-2 upon starvation, similar to that of Y27632 treatment ( Fig. 5b , lane 3). In contrast, the association of Bcl-2 with the T119E Beclin1 mutant was barely detectable upon nutrient stress because of a phospho-mimetic effect of the mutant ( Fig. 5b , lane 4). To confirm that T119 phosphorylation required for Bcl-2 dissociation was ROCK1 dependent, we examined Bcl-2 association of WT and T119A Beclin1, in the presence and absence of Y27632. As shown in Fig. 5c , Bcl-2 could not dissociate from Beclin1 T119A mutant and this was not further affected by the addition of ROCK inhibitor, Y27632. All of these results indicate that ROCK1 phosphorylation of Beclin1 at Thr119 is important for Bcl-2 dissociation. To further understand the importance of Beclin1 phosphorylation by ROCK1 in its dissociation from Bcl-2 during autophagy, we knocked down endogenous Beclin1 using siRNA towards the 3′-untranslated region, then ectopically expressed WT and mutant Beclin1 in these cells and examined LC3 processing. Consistent with the previous results, expression of Flag-Beclin1 WT induced higher levels of LC3II upon starvation, and this was inhibited upon Y27632 addition ( Fig. 5d ). However, Beclin1 T119A mutant-transfected cells had very low levels of LC3II upon metabolic stress and was not further affected by Y27632. In addition, WT and mutant-transfected cells were subjected to morphological analysis of LC3. Similar to the results from biochemical analysis ( Fig. 5 ), Flag-Beclin1 WT-transfected cells were able to induce LC3 punctae upon starvation. In addition, the treatment with Y27632 led to a significant decrease in endogenous LC3II ( Fig. 5e ). Of note, the Flag-Beclin1 T119A mutant showed impaired LC3 punctae formation, confirming true phospho-mutant activity. Consistently, the Flag-Beclin1 T119E ( Supplementary Fig. S11 ) mutant allowed cells to accumulate LC3 punctae at the autophagosomes, further confirming that phosphorylation of Beclin1 at Thr119 by ROCK1 is crucial for nutritional deprivation-mediated autophagy. ROCK1 deficiency causes defects in autophagy in vivo To determine whether ROCK1 has an important role in autophagy in vivo , we investigated starvation-induced autophagy in ROCK1 knockout (KO) mice. ROCK1 KO mice were generated using the Flp-Cre system ( Fig. 6a ). The KO was confirmed by genotyping and western blot analyses ( Fig. 6b , top and bottom panels, respectively). To monitor autophagy, levels of LC3II were evaluated in mice starved for 16 h. In ROCK1 KO hearts, the level of lipidated LC3 was markedly reduced as compared with that of starved Wt mice ( Fig. 6c and Supplementary Fig. S12a ). In addition, p62/SQSTM1, a scaffold protein known to be ubiquitinated and degraded via autophagy, accumulated at higher levels in ROCK1 KO hearts ( Fig. 6c ). As shown in Fig. 6d , it was possible to observe autophagosome structures in Wt starved tissue but not in ROCK1 KO mice. In addition, when cardiac muscle from starved mice were stained for the presence of endogenous LC3 punctae, there was a significant decrease in the LC3 puncta formation in ROCK1 KO mice ( Fig. 6e and Supplementary Fig. S12 ). Taken together, these results indicate that the loss of ROCK1 substantially impairs autophagy in vivo . 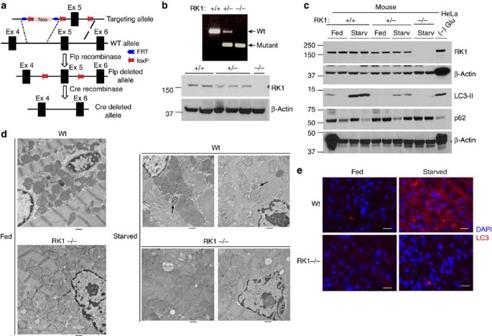Figure 6: Disruption of ROCK1 leads to impaired autophagyinvivo. (a) Genomic structure of ROCK1 (exon 4–6 only) with targeted allele, Flp-deleted allele and Cre-deleted allele. (b) PCR assay using tail genomic DNA from three different genotypes, separated on 0.7% agarose gel (top). Western blot analysis of ROCK1 expression in the heart tissue from three different genotypes using anti-ROCK1 antibody (bottom). β-Actin was used for protein loading control in each lane. (c) Mice were fed or starved for 16 h, and heart samples were prepared in lysis buffer. Resulting proteins were resolved by SDS–PAGE and blotted against ROCK1, LC3, autophagy marker p62 and β-actin. (d) ROCK1-deficient hearts or control hearts from animals fed or starved for 16 h were subjected to electron microscopy to identify autophagosome structures. Arrows indicate autophagic vacuoles. Scale bar, 500 nm. (e) Hearts from fed and starved ROCK1 WT and KO mice were sectioned, fixed in acetone and immunofluorescence assay was performed against endogenous LC3. Data are representative of two independent experiments from each genotype. Scale bar, 50 μm. Figure 6: Disruption of ROCK1 leads to impaired autophagy invivo . ( a ) Genomic structure of ROCK1 (exon 4–6 only) with targeted allele, Flp-deleted allele and Cre-deleted allele. ( b ) PCR assay using tail genomic DNA from three different genotypes, separated on 0.7% agarose gel (top). Western blot analysis of ROCK1 expression in the heart tissue from three different genotypes using anti-ROCK1 antibody (bottom). β-Actin was used for protein loading control in each lane. ( c ) Mice were fed or starved for 16 h, and heart samples were prepared in lysis buffer. Resulting proteins were resolved by SDS–PAGE and blotted against ROCK1, LC3, autophagy marker p62 and β-actin. ( d ) ROCK1-deficient hearts or control hearts from animals fed or starved for 16 h were subjected to electron microscopy to identify autophagosome structures. Arrows indicate autophagic vacuoles. Scale bar, 500 nm. ( e ) Hearts from fed and starved ROCK1 WT and KO mice were sectioned, fixed in acetone and immunofluorescence assay was performed against endogenous LC3. Data are representative of two independent experiments from each genotype. Scale bar, 50 μm. Full size image Using a proteomics approach, we identified ROCK1 as a vital factor during nutrient stress-induced autophagy. We showed further that Beclin1, an axial component of the autophagy machinery, is a substrate of ROCK1 when challenged with nutrient deprivation. The anti-apoptotic protein Bcl-2 serves as autophagy regulatory protein through its inhibitory association with Beclin1 (refs 16 , 19 ). Our results show that ROCK1 is activated during metabolic stress, leading to its increased binding and phosphorylation of the Beclin1 BH3 domain. We further demonstrate that metabolic stress-mediated ROCK1 phosphorylation of Beclin1 results in dissociation of Bcl-2 from the Beclin1 multiprotein complex without affecting UVRAG–Beclin1 interactions, and ultimately leads to autophagy ( Fig. 7 ). Consistent with an essential function of ROCK1 during the metabolic stress-mediated autophagy process in tissue culture cells, we demonstrated that the loss of ROCK1 function in mice substantially impairs autophagy during fasting. 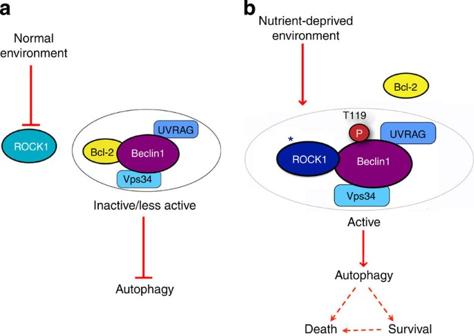Figure 7: A working model of ROCK1-mediated autophagy during nutrient stress. (a) Normal environment with sufficient glucose and nutrients suppresses ROCK1 activity. Bcl-2 thus associates with the Beclin1 core complex (Vps34 and UVRAG) and keeps autophagy in check. (b) When the cellular environment is deprived of nutrients, ROCK1 kinase is stimulated. ROCK1 binds and phosphorylates Beclin1 at T119 and disrupts Beclin1–Bcl-2 interaction. Dissociation of Bcl-2 triggers the Beclin1 core complex to induce autophagy and maintain a balance between cell survival and apoptosis. Figure 7: A working model of ROCK1-mediated autophagy during nutrient stress. ( a ) Normal environment with sufficient glucose and nutrients suppresses ROCK1 activity. Bcl-2 thus associates with the Beclin1 core complex (Vps34 and UVRAG) and keeps autophagy in check. ( b ) When the cellular environment is deprived of nutrients, ROCK1 kinase is stimulated. ROCK1 binds and phosphorylates Beclin1 at T119 and disrupts Beclin1–Bcl-2 interaction. Dissociation of Bcl-2 triggers the Beclin1 core complex to induce autophagy and maintain a balance between cell survival and apoptosis. Full size image The function of ROCK1 in membrane blebbing during apoptosis has been studied extensively [42] , [43] . We showed that impairment of ROCK1-mediated autophagy could lead to loss of cell viability under conditions of nutritional stress. These results imply that ROCK1 has additional roles to avoid cell death by providing energy in less severe, stressful circumstances. Thus, there appears to be an intricate balance of crosstalk between autophagy and apoptosis that is regulated by ROCK1 ( Fig. 7 ). Recently, other groups have also identified that ROCK1 regulates survival rather than apoptosis, under certain conditions [44] , supporting our results. However, it remains to be determined how ROCK1 kinase is activated under metabolic stress conditions. Several studies have shown that active RhoA-GTP binding to ROCK1 is required for ROCK1 activation [1] , [33] . However, we did not observe any increase in RhoA-GTP binding to ROCK1 upon nutritional stress, suggesting that other ROCK1-activating modulator(s), such as RhoE, may have a role. By mutational analysis, we localized Beclin1 Thr119 as the site of phosphorylation by ROCK1 upon starvation. This site is known to be a ROCK1 consensus motif, which is highly conserved among species, and is localized within the Beclin1 BH3 domain implicated in Bcl-2 binding [16] , [17] , [18] , [19] , [20] . We further demonstrated that Beclin1 phosphorylation at T119 by ROCK1 is crucial for the disassociation between Beclin1 and Bcl-2 during the autophagy upon metabolic stress. Recent reports suggest that DAPK (death associated protein kinase) also promotes autophagy via several different mechanisms [40] , [45] , [46] , [47] . DAPK has also been reported to phosphorylate Beclin1 in vitro at T119, resulting in the loss of interaction with Bcl-XL, but whether this mechanism is involved in nutritional stress-mediated autophagy has not been determined [40] . It is known that ROCK1 and DAPK share a consensus motif, R/KX/S/T or R/KXXS/T, for target phosphorylation [48] and share some common substrates, such as ZIPK [49] , [50] . Thus, each may phosphorylate Beclin1 under particular conditions. Nonetheless, our results suggest that ROCK1 is the major kinase responsible for phosphorylating Beclin1 at T119 and subsequently promoting the progression of autophagy during starvation. In this study, ROCK1-mediated phosphorylation of Beclin1 during nutrient stress leads to the induction of autophagy. However, ROCK1 may modulate autophagy through alternate mechanisms during nutrient stress. For example, ROCK1 was previously shown to activate the JNK pathway through JNK interacting protein (JIP-3) phosphorylation [5] , and upon nutrient deprivation activated JNK phosphorylates Bcl-2, resulting in the dissociation of Bcl-2 from Beclin1 and subsequent activation of autophagy [51] . Therefore, ROCK1 may modulate autophagy, not only through Beclin1 phosphorylation but concomitantly through ROCK1-mediated JNK activation, where these two arms essentially disrupt the Beclin1–Bcl-2 association and promote autophagosome formation. Further studies are needed to elucidate additional mechanisms by which ROCK1 regulates autophagy. ROCK1-induced autophagy may have critical functions in physiological and pathological contexts. Recent data suggests that Bcl-2-regulated autophagy during exercise is necessary to maintain glucose homeostasis in the muscle. However, previously known kinase phosphorylation of Bcl-2, such as JNK and mitogen-activated protein kinase, do not seem to have a role in this process [52] . Possibly, ROCK1-mediated phosphorylation of Beclin1, as shown here, could be important for Bcl-2-regulated autophagy during exercise. Although, ROCK1 and Beclin1 are well conserved among species, both genes are mutated in several human cancers [23] , [24] , [27] , [28] , [29] . Activating mutations of ROCK1 suggest a positive role for ROCK1 during cancer progression [30] , [44] . Accumulating evidence strongly suggest that autophagy may not only promote cancer cell survival but may also lead to chemoresistance [53] , [54] , [55] , [56] . As ROCK1 has a central role in autophagy and may promote cancer progression, inhibiting ROCK1 activity in cancer cells, in addition to chemotherapy, may help improve prognosis for cancer patients. Taken together, our data outlines a novel regulatory mechanism in which ROCK1 has an essential role during metabolic stress-induced autophagy. Cell lines and plasmids HeLa (human cervical cancer cells), EJ (human bladder cancer cells), 293T (human embryonic kidney cells) and IMR90 (normal human fibroblasts) cells were cultured in DMEM (CellGro) containing 10% fetal bovine serum (Invitrogen, CA), 100 U ml −1 penicillin and 100 μg ml −1 streptomycin at 37 °C. Where indicated, the cells were incubated in HBSS (CellGro) containing 10 mM HEPES-KOH (pH 7.5). The complementary DNA encoding Beclin1 was obtained from Open Biosystems (Clone: 2901072). Full-length Beclin1 (1–242) was then cloned into pcDNA3.1–Flag by PCR, using standard procedure. Mutagenesis in full-length Beclin1 (T119A, T119D and T119E) was performed using the megaprimer method. The obtained clones were sequenced in entirety to ensure no additional mutations were introduced during the PCR mutagenesis process. Flag-Beclin1 fragments (1–242,151–41 and 243–450) were obtained from Addgene [57] . Mutagenesis of Flag-Beclin1 1–242 fragment to obtain S22A, T38A and T119A was performed by similar method as detailed above. pEGFPC1-LC3 is described elsewhere [37] . Antibodies and reagents Antibodies used in this study are as follows: ROCK1 (IP: C19; WB: H85 (1:2,000); IF: K18 (1:700), Santa Cruz), ROCK2 (H85 (1:2,000), Santa Cruz), Beclin1 (IP: K15, Santa Cruz; WB: 3,495 (1:2,000), Cell Signaling; IF: 55,556 (1:700), Novus), PDI (3,501 (1:1,000), Cell Signaling), Mek1/2 (M17030 (1:1,000), Transduction Laboratories), Flag (M2 (1:200–1:500), Sigma), LC3 (3,868 (1:1,000), Cell Signaling), p-MYPT1 (04-773 (1:500), Millipore; 5,163 (1:500), Cell Signaling), MYPT1 (2634 (1:1000), Cell Signaling), p-Ser/Thr (22A, (1:250-5% milk) BD Biosciences), p62 (5114, (1:1,000), Cell Signaling), P -T119 Beclin1 (AP3765a (1:400), Abgent), β-actin (A5441 (1:10,000), Sigma), and DAPI (4′,6-diamidino-2-phenylindole) (1:10,000, Roche). Bafilomycin A1 (Sigma) was dissolved in dimethylsulphoxide, and Y27632 (Calbiochem) was dissolved in water. Complete protease inhibitor and PhosStop phosphatase inhibitor cocktail tablets were purchased from Roche. For cDNA and siRNA transfection, Lipofectamine 2000 (Invitrogen) and X-tremeGENE (Roche), respectively, was used according to manufacturers’ protocols. Immunoblot and IP For endogenous ROCK1 and Beclin1 IP, Crosslink IP kit (Thermo Pierce) was used according to the manufacturer’s recommendation with a few changes. In short, ROCK1 or Beclin1 antibody was crosslinked to Protein A/G agarose (Santa Cruz) using 450 μM disuccinimidyl suberate. Cells were lysed with the provided IP lysis buffer (0.025 M Tris, 0.15 M NaCl, 0.001 M EDTA, 1% NP-40, 5% glycerol; pH 7.4) supplemented with protease and phosphatase inhibitors (Roche), incubated on ice for 1 h, passed through a syringe and then centrifuged. Normalized lysates were mixed with ROCK1- or Beclin1-conjugated beads overnight, washed 4 × with 0.2% lysis buffer, followed by elution for 15 min at room temperature (RT). Flag IP was performed according to the manufacturer’s protocol and precipitated proteins were eluted using elution buffer (Thermo Pierce). Myc-IP was performed using Myc-conjugated agarose from Cell Signaling (3,400). For immunoblot analysis, cells were lysed with 1% Triton X-100 (v/v) lysis buffer (0.02 M Tris, 0.005 M EDTA, 0.01 M Na 4 P 2 O 7 , 0.1 M NaF, 0.002 M Na 3 VO 4 and 1% Triton X-100) with protease/phosphatase inhibitor cocktail, resolved by NuPAGE (Invitrogen) gels and transferred onto nitrocellulose membrane for detection with antibodies. Subcellular fractionation was performed as described previously [58] . Full-length images of immunoblots are shown in Supplementary Figs S13 and S14 . Immunofluorescence For ROCK1 and Beclin1 fluorescence, cells were grown on glass coverslips, subjected to glucose starvation and fixed with cold methanol for 10 min. Fixed cells were washed 3 × with 0.1% PBS–Triton X-100, blocked with 5% BSA-1% calf serum-containing PBS–Triton X-100 for 1 h at RT and incubated with primary antibodies (1:700 each) overnight. Staining was visualized with Alexa Fluor secondary antibodies using the Nikon A1 confocal microscope. For LC3 staining, cells on coverslips were cultured in DMEM or HBSS for indicated times. Cells were then washed in ice-cold PBS and fixed in chilled acetone for 5 min. LC3 puncta were labelled with anti-LC3B and counterstained with DAPI. For EJ cells stably transfected with GFP-LC3, treated cells were fixed in 2% paraformaldehyde for 10 min at RT. Cells were then washed extensively to remove any debris, counterstained with DAPI and examined using Zeiss VivaTome microscope. Förster resonance energy transfer HeLa cells were transfected with pZsYellow1-C1 (Clonetech-632444)-ROCK1 (cloned using Sac I and Sac II restriction enzyme sites) and mCER (Addgene-15214)-Beclin1 (cloned using Eco RI and Bam HI). For simplicity purpose, pZsYellow1-C1-ROCK1 was addressed as YFP-ROCK1 and mCER-Beclin1 as CFP-Beclin1. Transfected cells were plated on a glass bottom petri dish (Fluorodish, World Precision Instrument, Inc., Sarasota, FL) and maintained in normal (+glucose) DMEM media before switching to starvation (HBSS) media. Cells were placed on a Nikon Eclipse-Ti confocal microscope system equipped with an oil immersion × 60 numerical aperture 1.49 apo-TIRF objective, perfect focus and an environmental control incubation chamber (37 °C, 5% CO2). The emission fluorescence intensities were determined at 540±15 nm (YFP) and 482±18 nm (CFP) with a high-speed resonant scanner (dichroic mirror 457/514). The FRET ratio analysis was performed as previously described [59] . The FRET ratio was corrected for both the bleed-through of CFP into the 540 nm channel and the cross-talk due to the direct YFP excitation by light at 440 nm. Control experiments were performed with single fluorophore-transfected cells maintained in DMEM with high glucose. Media was changed to HBSS by perfusion, just as in FRET experiments. Protein purification and in vitro kinase assay For recombinant Beclin1, bacterial expression construct, pRSET, containing His-Beclin1 (full-length), was transformed in Escherichia coli BL21. Cells were induced with 1 mM isopropylthiogalactoside at 30 °C for 2 h. Cell pellet was resuspended in cold PBS and subjected to ultrasonication. Protein was purified using TALON beads (Clonetech) following the manufacturer’s protocol. In vitro kinase assay was performed using His-Beclin1 as substrate and recombinant ROCK1 (Millipore). HeLa cells were transiently transfected with Flag-Beclin1 constructs using Lipofectamine 2000. Thirty-six hours post transfection, cells were collected in lysis buffer supplemented with protease inhibitors. IP with Flag-agarose was performed and washed, and the resulting immune-complexed beads were used as substrate for the in vitro kinase assay. For in vitro kinase assay, recombinant MYPT1 (12–421, Millipore) or recombinant His-Beclin1 or Flag-Beclin1 constructs were used as substrates. Endogenous ROCK1 (immunoprecipitated from EJ cells) or recombinant ROCK1 was used as the kinase as indicated in figure legends. The kinase assay was performed as previously described [5] . In short, the substrate and kinase were incubated in kinase buffer (20 mM Tris, pH 7.5, 5 mM MgCl 2 , 100 mM KCl, 0.1 mM dithiothreitol, 100 μM ATP, 1 mM EDTA, 1 μM microcystin-LR, and 1 μCi [ 32 P]ATP) at 30 °C for 40 min. Reaction was terminated using SDS loading buffer, and proteins were resolved on 4–12% gel (NuPAGE), dried and exposed to film overnight at −80 °C. Electron microscopy Tissues were fixed in 2.0% glutaraldehyde in 0.1 M sodium cacodylate buffer, pH 7.4 (Electron Microscopy Sciences, Hatfield, PA) overnight at 4 °C. They were rinsed in buffer, post-fixed in 1.0% osmium tetroxide in cacodylate buffer for 1 h at room temperature, rinsed in buffer again and dehydrated through a graded series of ethanol to 100%. They were then infiltrated with Epon resin (Ted Pella, Redding, CA) in a 1:1 solution of Epon:ethanol. The following day, they were placed in fresh Epon for several hours and then embedded in Epon overnight at 60 °C. Thin sections were cut on a Leica EM UC7 ultramicrotome, collected onto formvar-coated grids, stained with uranyl acetate and lead citrate, and examined in a JEOL JEM 1011 transmission electron microscope at 80 kV. Images were collected using an AMT digital imaging system (Advanced Microscopy Techniques, Danvers, MA). Cells were fixed in the same glutaraldehyde fix for 1 h at room temperature. They were rinsed, scraped and pelleted, and osmicated as above. After further buffer rinses, they were embedded in 2.0% agarose for ease of handling and were dehydrated, infiltrated and embedded in Epon. Mice strains and tissue isolation The Rock1 allele in these animals contains loxP sites flanking exon 5 as described [60] . The floxed mice ( Rock1 flox/flox ) were bred with EIIa-cre mice to generate mice heterozygous for Rock1 exon 5 deletion ( Rock1 flox/− ). Rock1 flox/− heterozygous mice were then intercrossed to generate Rock1 −/− homozygous mice, designated as ROCK1 KO mice. All animals were housed in a temperature-controlled environment with 12-h light/dark cycles and ad libitum access to food and water. For starvation studies, male mice (8 weeks of age) were deprived of food for 16 h in clean cages but they received water ad libitum . ROCK1 (+/+) and ROCK1 (+/−): n =6 (fed) and n =5 (starved); ROCK1 ( −/− ): n =3 (fed) and n =3 (starved) mice were used. Experimental mice were killed by cervical dislocation, and the hearts were collected immediately and processed for immunofluorescence (washed in PBS and placed in OCT mounting medium) or frozen in liquid nitrogen for molecular analysis. These tissue samples were then lysed in lysis buffer using a Tissue Lyser on ice for 2 min. Protein was measured using Bradford, normalized and resolved on SDS–PAGE. All animal experiments were approved by the Subcommittee on Research Animal Care of Massachusetts General Hospital (protocol number2005N000022). How to cite this article: Gurkar, A. U. et al . Identification of ROCK1 kinase as a critical regulator of Beclin1-mediated autophagy during metabolic stress. Nat. Commun. 4:2189 doi: 10.1038/ncomms3189 (2013).